The global distribution of the Duffy blood group Blood group variants are characteristic of population groups, and can show conspicuous geographic patterns. Interest in the global prevalence of the Duffy blood group variants is multidisciplinary, but of particular importance to malariologists due to the resistance generally conferred by the Duffy-negative phenotype against Plasmodium vivax infection. Here we collate an extensive geo-database of surveys, forming the evidence-base for a multi-locus Bayesian geostatistical model to generate global frequency maps of the common Duffy alleles to refine the global cartography of the common Duffy variants. We show that the most prevalent allele globally was FY*A , while across sub-Saharan Africa the predominant allele was the silent FY*B ES variant, commonly reaching fixation across stretches of the continent. The maps presented not only represent the first spatially and genetically comprehensive description of variation at this locus, but also constitute an advance towards understanding the transmission patterns of the neglected P. vivax malaria parasite. First described 60 years ago in a multiply transfused haemolytic patient who lent his name to the system [1] , the Duffy blood group has since been of interest in diverse fields from anthropology [2] to genetics [3] and malariology [4] , [5] . Being of only occasional clinical significance [6] , much of the research into this weakly immunogenic blood group has been concerned with establishing characteristic expression patterns among populations. Easily diagnosable, the Duffy blood group quickly became part of the package of commonly investigated blood groups used to characterize the world's populations [7] and assess relatedness between communities. Interest in the Duffy blood group rose substantially, however, following experimental demonstration of the malaria parasite Plasmodium vivax 's dependency on the Duffy antigen for establishing erythrocytic infection [8] , [9] , [10] , and therefore that erythrocytes lacking the antigen were refractory to this parasitic infection. This Duffy negativity phenotype, long known to be common among sub-Saharan African populations [11] , provided an explanation for the apparent absence of P. vivax among these populations and their diaspora [12] . To date, no other erythrocyte receptor has been described for P. vivax , although some cases of infection have been reported in Duffy-negative individuals [13] , [14] , [15] . Furthermore, the universal expression of the Duffy antigen binding protein ( Pv DBP) has made this merozoite invasion ligand protein a prime P. vivax vaccine target [16] . The role of the Duffy receptor in P. vivax infection, therefore, allows the Duffy-negative phenotype to be a proxy of host resistance to blood stage infection [17] . Recognizing its physiological function as a chemokine receptor involved in inflammation, the Duffy antigen is also known as the Duffy antigen receptor for chemokines (DARC). Although specific mechanisms underlying its functions remain uncertain, there is interest in DARC as an explanatory variable for population-specific differences in disease susceptibility [18] , as demonstrated by ongoing research into its role in inflammation-associated pathology and malignancy [18] , [19] , and the recent, though highly controversial [20] , surge in interest around the antigen's role in HIV infection [21] . The monogenic Duffy system was the first human blood group assigned to a specific autosome: position q21–q25 on chromosome 1 (ref. 22 ). The gene product has two main variant forms: Fy a and Fy b antigens, which differ by a single amino acid (Gly42Asp), encoded by alleles FY*A and FY*B , which are differentiated by a single base substitution (G125A) [23] , [24] . Duffy expression is disrupted by a T to C substitution in the gene's promoter region at nucleotide −33, preventing transcription and resulting in the null 'erythrocyte silent' (ES) phenotype. This promoter-region variant is commonly haplotypically associated with the FY*B coding region (corresponding to the FY*B ES allele) [24] , although occasional reports of association with the FY*A sequence have been published ( FY*A ES allele) [25] , [26] . These four alleles combine to ten possible genotypes ( Fig. 1 ), with FY*A and FY*B alleles expressed codominantly over the null variants FY*B ES and FY*A ES . Genotypes therefore correspond to four phenotypes: Fy(a+b+), Fy(a+b−), Fy(a−b+) and Fy(a−b−). Further details about the genetics and molecular aspects of the Duffy system, including other rare variants such as the weakly expressed FY*X allele [27] (expressed as the Fy(b+ weak ) phenotype), are fully discussed by Langhi and Bordin [23] and Zimmerman [24] . 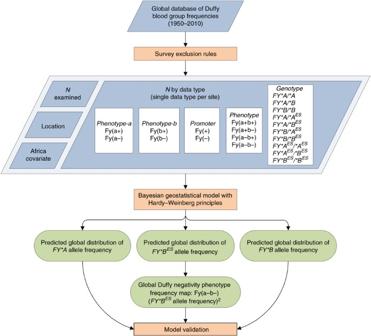Figure 1: Schematic overview of the procedures and methods. Blue diamonds describe input data. White boxes within the 'Nby data type' diamond represent different possible data types, with each spatially unique survey being represented by only one white box. Orange boxes denote models and experimental procedures. Green rods indicate model outputs. Figure 1: Schematic overview of the procedures and methods. Blue diamonds describe input data. White boxes within the ' N by data type' diamond represent different possible data types, with each spatially unique survey being represented by only one white box. Orange boxes denote models and experimental procedures. Green rods indicate model outputs. Full size image The common Duffy alleles present striking patterns of geographic differentiation, which have only once been mapped spatially, as part of Cavalli-Sforza et al . 's [28] efforts to unravel the genetic history of human populations. Alleles were mapped in isolation of each other ( FY*A , FY*B and FY*B ES ) using limited subsets of data which directly informed the frequency of each particular variant. Previous methodology, which used a sequential inverse distance weighting algorithm, was unable to estimate uncertainty in the mapped predictions. Since this publication in 1994, new data have been generated, much of which have benefitted from full genotyping. In addition, significant advances have been made to geostatistical mapping techniques allowing more rigorous predictions of spatially continuous variables using data obtained at a limited number of spatial locations [29] , and varied data inputs to inform all output predictions simultaneously. Here we first assembled an updated data set based on a thorough review of published and unpublished data, then used this to generate global maps of the Duffy alleles and the Duffy negativity phenotype using a bespoke Bayesian geostatistical model. This generated for every location on a gridded surface a posterior distribution of all predicted values from the model's thousands of iterations, representing a complete model of uncertainty from which median values were derived to generate point-estimate maps. In addition to providing fundamental biomedical descriptions of human populations with potential applications for explaining population-level variation to a range of clinical conditions [19] , these maps are intended to support contemporary analyses of P. vivax transmission risk [17] . The survey database Literature searches identified 821 spatially unique data points of Duffy blood type prevalence matching the database inclusion criteria for representativeness ( Supplementary Data ). These represented a total of 131,187 individuals sampled, 17.8% of whom were surveyed on the African continent ( Table 1 ). Of this total, 536 surveys were geopositioned as points (≤25 km 2 ), and 285 mapped as polygon centroids. Polygons were digitized and centroid coordinates calculated in GIS software (ArcView GIS 3.2 and ArcMap 9.3, ESRI). Surveys reported only to province or country level were considered to lack sufficient geographical specificity and were thus excluded. A total of 89 additional data points were excluded, as they could not be located with sufficient precision. The selected data points were relatively evenly distributed between regions, with 32% in the Americas, 25% in Africa, 26% in Asia and 17% in Europe ( Fig. 2 ). Survey sample sizes were highly variable: ranging from 1 to 2,470. The mean size was 160 and the median 99. Table 1 Summary of input data. 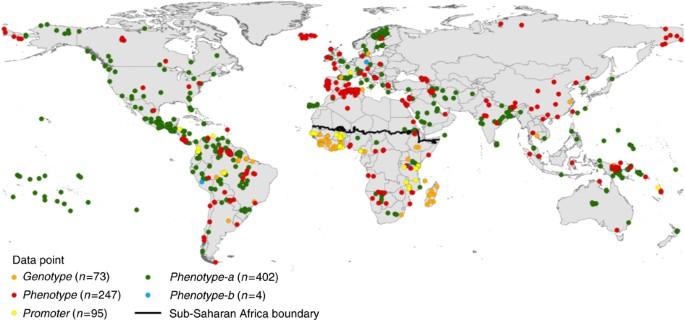Figure 2: Spatial distribution of the input data points categorized by data type. Symbol colours represent the type of information in the survey: orange when full genotypes were detected (Genotype); red for full phenotype diagnosis (Phenotype); yellow for expression/non-expression of Duffy antigen (Promoter); green and blue for partial phenotypic data, about expression of Fya(Phenotype-a) and Fyb(Phenotype-b) respectively. Total data points aren=821; totals by data type are listed in the legend. The sub-Saharan Africa covariate boundary is shown in black. Full size table Figure 2: Spatial distribution of the input data points categorized by data type. Symbol colours represent the type of information in the survey: orange when full genotypes were detected ( Genotype ); red for full phenotype diagnosis ( Phenotype ); yellow for expression/non-expression of Duffy antigen ( Promoter ); green and blue for partial phenotypic data, about expression of Fy a ( Phenotype-a ) and Fy b ( Phenotype-b ) respectively. Total data points are n =821; totals by data type are listed in the legend. The sub-Saharan Africa covariate boundary is shown in black. Full size image Serological techniques were the only methods used for blood typing until the 1990s, ( Supplementary Fig. S1 ). Half of the surveys (49%) used anti-Fy a antiserum only, thus were recorded as ' Phenotype-a ' data types (402 of 821 surveys). Complete ' Phenotype' data were provided in 247 surveys (30%). Molecularly diagnosed ' Genotype ' and ' Promoter ' data (9 and 12%, respectively) were only commonly reported in post-2000 surveys, and mainly across Africa (71% of the 168 DNA-based records were from Africa). The five categories of data types are summarized in Table 2 , and the spatial distribution of each is represented by the colour-coded data point map in Figure 2 . Relative proportions of each variant-type reported by data type and continent are displayed in Table 1 ; further summaries of the data are presented graphically by decade in Supplementary Figures S1-S2 . Table 2 Diagnostic methods and corresponding classification data type categories. Full size table The maps To generate continuous global maps from the assembled database, a Duffy-specific geostatistical model was developed ( Supplementary Methods ). Its key features are as follows: first, to incorporate all genotypic variants and data types simultaneously; second, to predict any genotype or phenotype frequency desired; third, to allow for local heterogeneity; and fourth, to take into account sampling error through sample size, while also generating uncertainty estimates with the prediction at each spatial unit (pixel). Allele frequencies Continuous global frequency maps of each of the three common Duffy alleles ( FY*A , FY*B and FY*B ES ) were generated simultaneously, along with summaries of uncertainty in the predictions quantified by the 50% interquartile range (IQR; Fig. 3 ). Full statistical summaries of the model parameters at each locus are provided in Supplementary Table S1 . The silent FY*A ES allele could not be modelled spatially due to its rarity (see Methods). 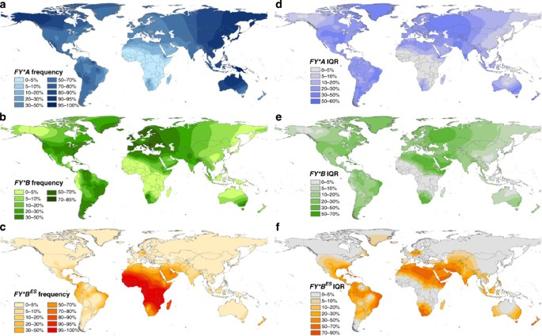Figure 3: Global Duffy blood group allele frequencies and uncertainty maps. (a–c) Correspond toFY*A,FY*BandFY*BESallele frequency maps, respectively (median values of the prediction posterior distributions); (d–f) show the respective interquartile ranges (IQR) of each allele frequency map (25–75% interval). Predictions are made on a 5×5 km grid in Africa and 10×10 km grid elsewhere.Supplementary Figure S5is a greyscale image of this figure. Figure 3: Global Duffy blood group allele frequencies and uncertainty maps. ( a – c ) Correspond to FY*A , FY*B and FY*B ES allele frequency maps, respectively (median values of the prediction posterior distributions); ( d – f ) show the respective interquartile ranges (IQR) of each allele frequency map (25–75% interval). Predictions are made on a 5×5 km grid in Africa and 10×10 km grid elsewhere. Supplementary Figure S5 is a greyscale image of this figure. Full size image The allele frequency maps reveal strong geographic patterns, the most conspicuously focal being the distribution of the silent FY*B ES allele across sub-Saharan Africa. Allelic frequencies across 30 countries in this region are characterized by >90% FY*B ES and frequencies of 0–5% for FY*A and FY*B ( Fig. 3a–c ). Frequencies indicate fixation (that is, frequencies of 100% (ref. 30 )) in parts of west, central and east Africa, suggesting total refractoriness of the local population to P. vivax infection [3] , [30] . The FY*B ES allele, however, is not confined to the mainland African sub-continent, with frequencies predicted above 80% across Madagascar and above 50% through the Arabian Peninsula ( Fig. 3c ). Low allelic frequencies have also spread into the Americas, notably along the Atlantic coast and in the Caribbean. Median frequencies of 5–20% are predicted across India and up to 11% in South-East Asia. Allelic heterogeneity is greatest in the Americas, with all three alleles predicted as being present and with only localized patches of predominance of single alleles. The FY*A allele ( Fig. 3a ) is close to fixation across pockets of eastern Asia, and remains high with median frequencies above 80% predicted across large extents of south Asia, Australia and in populations from Mongolia and eastern parts of China and Russia. The allele is also at high frequencies (>90%) in Alaska and northwest Canada. Outside these regions of highest predominance, FY*A remains relatively common outside the African continent, with median frequencies >50% predicted across 67.7% of the global surface. The FY*B allele ( Fig. 3b ) is the allele least prevalent globally, with a maximum predicted median frequency of 83% (thus fixation is never reached). Reflecting its reduced prevalence, the distribution of FY*B matches areas of highest allelic heterogeneity, where its presence increases to frequencies similar to, or greater than, FY*A and FY*B ES . Frequencies above 50% are restricted to Europe and pockets of the Americas, notably along the east coast of the United States of America. FY*B frequencies decrease from their European epicentre eastwards, as the FY*A allele becomes predominant in Asia. FY*B is also prevalent in the buffer zones around the region of FY*B ES predominance, in northern, north-eastern and southern Africa. Duffy negativity phenotype The phenotype map of Duffy negativity ( Fig. 4 ) reveals very low frequencies of the homozygous null genotype ( FY*B ES /*B ES ) from much of the predicted non-African FY*B ES distribution ( Fig. 3c ). Despite being present, the low allelic frequencies mean that homozygotic inheritance is too low to feature in the phenotype map. Therefore, even more pronounced than the allele's distribution, the Duffy negativity phenotype is highly constrained to sub-Saharan African populations, and localized patches in the Americas. Across the African continent, the phenotype's median frequency is greatest (98–100%) in western, central and south-eastern regions from The Gambia to Mozambique, buffered by a high median frequency region of ≥90% frequency covering 22 countries ( Fig. 4a ). Around this high frequency region, steep clines into the Sahel in the north, and Namibia and South Africa in the south lead to median phenotypic frequencies of <10% in parts of these extremities. 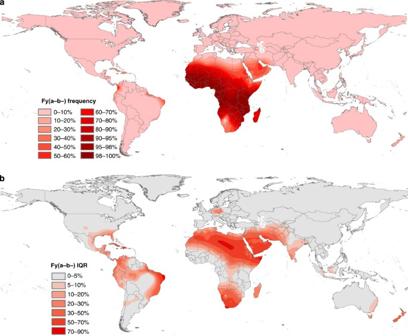Figure 4: Global distribution of the Duffy negativity phenotype. (a) Global prevalence of Fy(a−b−); (b) associated uncertainty map. Uncertainty is represented by the interval between the 25 and 75% quartiles of the posterior distribution (IQR).Supplementary Figure S6is a greyscale image of this figure. Figure 4: Global distribution of the Duffy negativity phenotype. ( a ) Global prevalence of Fy(a−b−); ( b ) associated uncertainty map. Uncertainty is represented by the interval between the 25 and 75% quartiles of the posterior distribution (IQR). Supplementary Figure S6 is a greyscale image of this figure. Full size image Frequencies of Duffy negativity increase by ∼ 10% south of the sub-Saharan desert boundary, as defined in the model by the GlobCover bare ground data set [31] ( Fig. 5 ). This trend of increased frequencies is reflected by the positive values associated with the sub-Saharan Africa covariate, fully described in Supplementary Table S2 . The increase is sharpest where there are few underlying data points, contrasting with the prediction in data-rich regions, such as West Africa, which is smoother across the desert boundary due to the abundance of input data overriding its influence. 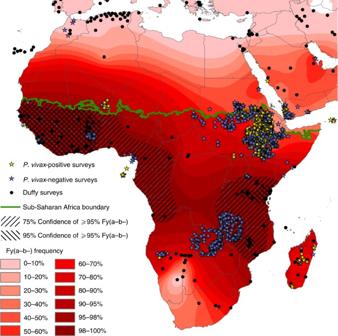Figure 5: Characteristics of the Duffy negativity phenotype in Africa. This figure shows the covariate line (in green), which separates sub-Saharan African populations from the rest of the continent; hatched areas indicate areas of confidence in the distribution of ≥95% Duffy negativity frequency: with 75%and 95% confidence. Black data points correspond to the input Duffy data points (n=821). Yellow stars indicate locations ofP. vivax-positive community surveys (n=354), and blue starsP. vivax-negative surveys (n=1405) (data assembled by the Malaria Atlas Project17,46).Supplementary Figure S7is a greyscale image of this figure. Figure 5: Characteristics of the Duffy negativity phenotype in Africa. This figure shows the covariate line (in green), which separates sub-Saharan African populations from the rest of the continent; hatched areas indicate areas of confidence in the distribution of ≥95% Duffy negativity frequency: with 75%and 95% confidence. Black data points correspond to the input Duffy data points ( n =821). Yellow stars indicate locations of P. vivax -positive community surveys ( n =354), and blue stars P. vivax -negative surveys ( n =1405) (data assembled by the Malaria Atlas Project [17] , [46] ). Supplementary Figure S7 is a greyscale image of this figure. Full size image Prediction uncertainty The output generated by the Bayesian framework is a predictive posterior distribution for each modelled variable for each 10×10 km pixel on the global grid (and 5×5 km across Africa). The posterior quantifies the probabilities associated with every candidate value of each modelled variable and therefore represents a complete description of uncertainty in the model output [32] . The outputs, summarized in Figures 3a–c and 4a , are the median values of these distributions. The uncertainties around these predictions, represented by the intervals between the 25 and 75% quartiles of the posterior distributions (or IQRs), are shown for the allele maps in Figures 3d–f and for Duffy negativity in Figure 4b . Remarkable certainty in the prediction for high Duffy negativity in sub-Saharan Africa is reflected by IQRs of 0–5% for all outputs. The absence of data points from the Democratic Republic of the Congo leads to a slightly elevated level of uncertainty relative to the surrounding region ( Figs 4b and 5 ). Certainty in the prediction of the highest frequencies of Duffy negativity is illustrated by the hatched areas of ≥95% Duffy negativity prevalence, determined with 75 and 95% confidence ( Fig. 5 ). As would be expected from the heterogeneity in allelic make-up ( Fig. 3a,b ), the greatest uncertainty in the global predictions of FY*A and FY*B prevalence is associated with the predictions across Europe, western Asia and the Americas ( Fig. 3d,e ). Validation statistics Bespoke validation procedures were developed to quantify the model's ability to predict frequencies of each allele, as well as the validity in the underlying assumption of Hardy–Weinberg equilibrium: first, by validating the Duffy-negative phenotype surface; second, by assessing rates of heterozygosity between FY*A and FY*B . The model's predictive ability was quantified by assessing the disparity between model predictions and held-out subsets of data excluded for validation analyses [33] . The validations were summarized using simple statistical measures: mean error (assesses overall model bias) and mean absolute error (quantifies overall prediction accuracy as the average magnitude of the errors, Supplementary Methods ). First, the mean error in the prediction of the Duffy negativity phenotype revealed a slight positive bias in the posterior predictive distribution of Duffy negativity (mean error: 1.3%), while the mean absolute error revealed relatively high typical precision in the predictions (mean absolute error: 5.8%). Second, the heterozygosity validation process identified an overall positive bias in the posterior predictive distribution of rates of heterozygosity (frequencies of the FY*A/*B genotype) with mean error of 5.5% and mean absolute error of 7.8%. Overall, therefore, the model's predictive ability for the clinically significant Duffy-negative phenotype was relatively high, although the assumption of Hardy–Weinberg equilibrium was not strongly supported, indicating that better predictions might be achieved in future iterations by modelling the fixation index as a third geostatistical random field. However, the resulting model would be substantially more complicated than the current one, which is already a major advance beyond the state of the art, and commensurately more difficult to fit. Given the relatively small size of the heterozygote deficiency in the holdout data set, we decided against elaborating the model in the current study. More validation results are given in Supplementary Figure S3 . The spatial distribution of the Duffy blood group variants has been of interest since its discovery 60 years ago because of its link to the pathology of both infectious and non-communicable diseases, including most notably with P. vivax infection. We have assembled an up-to-date database of Duffy phenotypic and genotypic data, from which we identified 821 geographically unique community surveys, and developed a geostatistical model to generate global frequency maps for the main Duffy alleles, as well as the first map of the Duffy-negative phenotype. These refined maps and associated uncertainty measures allow both an assessment of the quality and distribution of existing data as well as a discussion of how the maps may help direct further research into the interactions between Duffy negativity and P. vivax malaria. A detailed comparison with the existing maps from Cavalli-Sforza et al . [28] is presented in the Supplementary Discussion and Supplementary Figures S8-S10 . The summary median maps presented reveal relatively smooth global-scale patterns of geographic differentiation among populations. Despite being considered the ancestral allele [34] , our maps show a remarkable restriction in the distribution and frequency of the FY*B allele, with highest prevalence found in Europe and parts of the Americas, with further patches of increased prevalence in areas buffering the region of FY*B ES predominance in sub-Saharan Africa. Frequencies of FY*A prevalence increase with distance from Africa and Europe, becoming dominant across south-east Asia, including those areas where P. vivax endemicity is highest [17] . Although the FY*B ES allele map predicts presence outside the African continent and the Arabian Peninsula, its frequencies remain too low for the Duffy-negative phenotype frequencies to exceed 10%. Although these static contemporary representations of allelic frequencies cannot alone be interpreted to advance current speculation regarding the causative mechanisms of selection of the high frequencies of the FY*B ES allele [4] , [5] , [35] , [36] , the Duffy negativity map does reflect visually the historical areas of malaria transmission, as defined by Lysenko's pre-control era malaria map [37] ( Supplementary Fig. S4 , recently republished by Piel et al . [38] ) A major challenge in this study was synthesizing the results of surveys, which used a range of diagnostic methods with potentially different reliabilities, particularly between genotyping and phenotyping methods. The possible influence of such variability on the model input is reviewed in detail in the Supplementary Methods , but is not considered to have major influence on the final output. By categorizing results into five data types ( Table 2 ) and developing a versatile geostatistical model, we were able to draw information from the differing data types in our full data set to generate each allele frequency map simultaneously. The Genotype data, generated from molecular diagnostic methods only widely available after the previous maps [28] were published, were most informative for the model. Despite a generally good global spread of survey data points ( Fig. 2 ), the uncertainty maps allow identification of areas where additional data would have proportionally greatest impact on our understanding of the distributions. Both the quality (data type) and quantity (data distribution) of the data affect the uncertainty measures. Uncertainty is increased by both scarcity of input data (exemplified across the Arabian Peninsula where only Phenotype-a data were available) and heterogeneity (characteristic of the Americas where populations of diverse origins coexist; Figs 3d–f and 5 ). In contrast, areas of lowest uncertainty match data-rich regions and areas of near-fixation, illustrated by the hatched areas of 95% confidence in the prediction shown in Figure 5 . Scarcity of input data also leaves us uncertain about possible fine-scale variation of allelic heterogeneity. This is demonstrated by the relatively high uncertainty in the predictions of the patchily distributed FY*B ES allele across the Americas, where spatial heterogeneity is expected to be high and perhaps not fully represented by the data set. As well as improving reliability in the current predictions, additional molecularly diagnosed data would allow refinements of the model to include additional polymorphic variants, such as the low-frequency weak FY*X variant [39] . This is discussed in detail in the Supplementary Discussion . Reflecting the growing appreciation of P. vivax 's public health significance and the realization that it is not 'benign' [16] , [40] , [41] , the parasite's relationship with the Duffy receptor is the primary focus of contemporary studies of the Duffy antigen. However, two lines of evidence, both from a community and an individual standpoint, support the need for further research into the Duffy–parasite association. First, contrary to expectation, there is evidence of P. vivax transmission in areas mapped with highest Duffy negativity frequencies. Although widespread surveys have failed to identify the parasite in this region (including a continental-wide survey by Culleton et al . [42] , and the data set of community parasite rate surveys displayed in Fig. 5 ), reports of infected mosquitoes [13] , travellers [17] and exposed individuals [43] suggest low level transmission. Across this predominantly Duffy-negative region, very low numbers of Duffy-positive individuals were identified (0.6% of individuals in 123 surveys across the 98–100% Fy(a−b−) region; Supplementary Table S3 ). To see whether these two observations can be reconciled to explain transmission, mathematical modelling is needed to estimate the basic reproductive number (R 0 ) of P. vivax (as done for Plasmodium falciparum [44] ) to help assess whether the very low predicted frequencies of susceptible Duffy-positive hosts could sustain transmission in populations mapped as predominantly Duffy negative. Second, from areas mapped with high Duffy phenotypic heterogeneity, P. vivax infections have been identified in Duffy-negative hosts (in Madagascar [15] and Brazil [14] ). If this phenomenon of infected Fy(a−b−) individuals is associated with local Duffy heterogeneity, as hypothesized by Ménard et al . [15] , the Duffy maps presented here could be used to target further studies in other heterogeneous P. vivax endemic areas [17] , including southern Africa, Ethiopia, southern Sudan and pockets of the Brazilian and Colombian coasts. Investigation of P. vivax transmission in these areas particularly, but also across regions with a spectrum of characteristic Duffy phenotypes, could provide vital public health insights into P. vivax populations at risk, particularly when coupled with host-level data on Duffy types. In this era of increasing concern about the P. vivax parasite, we believe that a contemporary spatial description of the prevalence of the Duffy antigen receptor is essential for optimizing our understanding of the parasite's clinical burden. The geopositioned database and maps represent a new effort to document the spatial characteristics of a fundamental biomedical trait implicated in haematological and other clinical contexts. The versatile geostatistical model developed was adapted to a multiple-locus trait, informed by a range of input data types to generate a suite of output products. Such methods are uncommonly used by the genetics community, but we believe could have an important role in the current era of large-scale spatial genomic analyses. Although we present a cartographic suite which we believe constitutes a significant improvement from previously published attempts [28] (see Supplementary Discussion and Supplementary Figs S8-S10 ), this study highlights limitations to our current knowledge of the Duffy blood group: both in terms of the scarcity of data from many areas, and in relation to the P. vivax invasion pathway. All collated data and model code will be made openly accessible. Analysis outline The methodological steps of this work were threefold: first, to assemble a library of full-text references describing Duffy blood group surveys, complemented with unpublished data; second, to abstract the Duffy frequency data from each source and to georeference survey locations; and third, to develop a spatial model which uses the full heterogeneous data set assembled to predict continuous global frequency maps of the Duffy variants. A schematic overview of the methodological process is given in Figure 1 , and each component is now discussed in more detail. Library assembly Systematic searches, adapted from those developed by the Malaria Atlas Project (MAP, http://www.map.ox.ac.uk ) [45] , [46] were conducted in an attempt to assemble a comprehensive database of Duffy blood group surveys dating from 1950, the publication year of Cutbush's description of the blood group [1] . Keyword searches for 'Duffy' and 'DARC' were conducted in online bibliographic archives PubMed ( http://www.pubmed.gov ), ISI Web of Knowledge ( http://isiwebofknowledge.com ) and Scopus ( http://www.scopus.com ). Searches were last performed on 08 December 2009. Manual duplicate removal and abstract reviews of the amalgamated search results identified 303 references likely to contain data, in addition to the 296 and 60 references from existing databases published by Mourant et al . [47] and Cavalli-Sforza et al . [28] , respectively. Full-text searches were then conducted for each of these 659 unique references. Following direct contact with researchers, 15 additional unpublished data sets were also included. All sources from which data met the criteria for inclusion are cited in the Supplementary References . Data abstraction and inclusion criteria The library of assembled references was reviewed to identify location-specific records of Duffy variant frequencies representative of local populations. Data were abstracted into a customized database, including population descriptions and ethnicities as reported by authors, methodological details and Duffy variant frequencies. Potentially biased samples of hospital patients with malaria symptoms or recently transfused individuals were excluded, as were family-based investigations and studies focussing on selected subgroups of larger mixed communities (for example, African-American communities in American cities). No constraints were placed on sample size, as the geostatistical framework downweighted the information content of very small surveys in accordance with a binomial sampling model [33] . Geopositioning The geographic location of each survey was determined as precisely as possible using the georeferencing protocol previously described by Guerra et al . [45] . Author descriptions of survey sites were used to verify locations identified in digital databases including Microsoft Encarta (Microsoft Corporation), and online databases such as Geonames (National Geospatial-Intelligence Agency, http://geonames.nga.mil/ggmagaz/ , accessed June–December 2009) and Global Gazetteer Version 2.2 (Falling Rain Genomics, http://www.fallingrain.com/world/index.html, accessed June–December 2009). Surveys were categorized according to the area they represented: points (≤25 km 2 ), and small (>25 and ≤100 km 2 ) or large polygons (>100 km 2 ). Duffy blood group data In addition to prevalence data of specific variants, details of diagnostic methodology were recorded to classify the type of information provided from the survey ( Table 2 ). According to the range of possible serological and molecular diagnostic methods, data points were classified into five data types: ' Genotype ', where full genotypes were reported; ' Phenotype ', if full serological diagnoses were performed (with both anti-Fy a and anti-Fy b antisera); ' Promoter ', if results reported only antigen expression/non-expression without distinguishing Fy a from Fy b (data were mainly from molecular studies examining only the promoter-region locus, but also occasionally from serological tests not distinguishing between antigenic variants); ' Phenotype-a ', if only the Fy a antigen was tested for (meaning that presence of Fy b antigen could not be distinguished from the negativity phenotype); and ' Phenotype-b ', if the study was only concerned with Fy b expression ( Fig. 6 ). 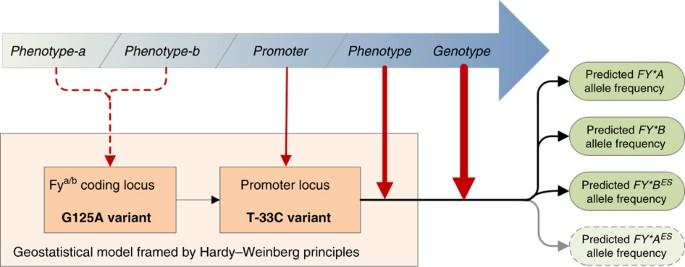Figure 6: Relationship between data types and the information conveyed to the model. Left to right along the large arrow, the deepening colour intensity represents each data type's relative influence on the model output. Dashed vertical arrows denote information about only one locus. Thickness of vertical lines emphasizes the completeness of the data type. Orange boxes represent the Bayesian model. Green rods indicate output data. The grey horizontal arrow and greyedFY*AESprediction rod indicates that this allele was accounted for in the model structure, but not one of the final outputs. Figure 6: Relationship between data types and the information conveyed to the model. Left to right along the large arrow, the deepening colour intensity represents each data type's relative influence on the model output. Dashed vertical arrows denote information about only one locus. Thickness of vertical lines emphasizes the completeness of the data type. Orange boxes represent the Bayesian model. Green rods indicate output data. The grey horizontal arrow and greyed FY*A ES prediction rod indicates that this allele was accounted for in the model structure, but not one of the final outputs. Full size image Modelling To accommodate the five input data types described and to model the multiallelic system, the two primary loci differentiating the Duffy variants were considered simultaneously. These were position −33 in the promoter region, which determines expression/non-expression, and base position 125 of exon 2, differentiating Fy a from Fy b coding regions [23] . Including the full data set while modelling each variant optimizes the model predictions, as each data type informs, either directly or indirectly, the frequency of variants at both loci, by ruling out certain genotypes. This feature was not possible with previously used mapping models [28] . Genetic loci modelled The genetic loci were considered as two spatially independent random fields, but modelled in association: first, the random field representing the coding region variant modelled the frequency of Fy a or Fy b expression; and second, a random field represented the probability of the promoter 'ES' variant being associated with the Fy b coding variant, thus determining prevalence of FY*B versus FY*B ES alleles. Reports in the data set of the 'ES' variant in association with the Fy a variant (that is, the FY*A ES allele) were too infrequent and, when identified, were too rare to be modelled as a spatial random field. Therefore, this variant was modelled by a small constant. Further details about the model are given in the Supplementary Methods . Sub-Saharan Africa covariate Preliminary examination of the ' Genotype ' data set confirmed the assumption that the haplotypic association between the Fy b coding variant and the 'ES' promoter variant, together corresponding to the FY*B ES allele, was very high within sub-Saharan African populations, but rare outside the region. To allow the model to reflect this high probability of association across sub-Saharan Africa, we used a generalized version of the GlobCover Land Cover V2.2 bare ground surface (channel 200) [31] to differentiate the sub-Saharan populations (presence), including those living in Madagascar and on other nearby islands (decision informed by the ' Genotype' data), from the other populations (absence; Fig. 2 ). This binary descriptor was the only covariate used in the model. Model implementation The analyses were implemented in a Bayesian model-based geostatistical framework [29] , the principal aspects of which have been previously described [33] , [48] . In brief, the geostatistical model uses Gaussian random fields to represent the spatial heterogeneity observed in the data and to predict values at unsampled locations. Repeated sampling of the random fields ensures that a representative sample of all the possibilities consistent with the input data set is used in predicting pixel values at sites where there is no data ( Supplementary Methods ). Estimates for pixels distant from any input data points or in areas of high spatial heterogeneity are inherently more difficult to predict precisely, and so are associated with greater prediction uncertainty. The posterior median values and associated uncertainty (IQR (25th to 75th percent quartile ranges) of the posterior distribution) are used to summarize the model's predictions for each pixel [33] , [49] . Generating the map surfaces The model's predictions for allele frequencies were mapped at all pixels on the global grid (at 5×5 km in Africa and 10×10 km elsewhere). Median values of the posterior distribution were chosen for the maps as these were considered more appropriate than mean values, due to the long-tailed distributions of the predictions that could strongly skew mean estimates. From these allele frequency surfaces, genotype frequencies could be obtained using the standard Hardy–Weinberg formula [50] , [51] . Thus, the Duffy negativity phenotype was expressed by the squared frequency of the silent FY*B ES allele (the FY*A ES allele being too rare to occur in homozygous form). Model validation To validate the three allele frequency surfaces and cross-examine the model's assumption of Hardy–Weinberg equilibrium, both the frequency of Duffy negativity and frequency of FY*A/*B heterozygosity were validated. For each validation procedure, the model was run with a random subset of the data set left out and predictions at these locations were compared with the observed frequencies. Estimates of the model's overall bias and precision were quantified as mean error and mean absolute error values, respectively ( Supplementary Methods ). Availability of data The survey database and maps are publicly accessible through the MAP website ( http://www.map.ox.ac.uk ) in line with the MAP's open-access policy and the terms of the Wellcome Trust Biomedical Resources Grant (#085406) funding this work. How to cite this article : Howes, R.E. et al . The global distribution of the Duffy blood group. Nat. Commun. 2:266 doi: 10.1038/ncomms1265 (2011).